The structure of apo-kinesin bound to tubulin links the nucleotide cycle to movement Kinesin-1 is a dimeric ATP-dependent motor protein that moves towards microtubules (+) ends. This movement is driven by two conformations (docked and undocked) of the two motor domains carboxy-terminal peptides (named neck linkers), in correlation with the nucleotide bound to each motor domain. Despite extensive data on kinesin-1, the structural connection between its nucleotide cycle and movement has remained elusive, mostly because the structure of the critical tubulin-bound apo-kinesin state was unknown. Here we report the 2.2 Å structure of this complex. From its comparison with detached kinesin–ADP and tubulin-bound kinesin–ATP, we identify three kinesin motor subdomains that move rigidly along the nucleotide cycle. Our data reveal how these subdomains reorient on binding to tubulin and when ATP binds, leading respectively to ADP release and to neck linker docking. These results establish a framework for understanding the transformation of chemical energy into mechanical work by (+) end-directed kinesins. In the cell, the main function of kinesin-1 (previously named conventional kinesin and hereafter called kinesin) is to transport organelles. It does so by moving processively towards the (+) end of microtubules, a process tightly coupled to the ATP hydrolysis cycle [1] . Kinesin consists of two identical motor domains connected by a coiled-coil stalk and a pair of light chains that bind to the tail C-terminal domains. The motor domain harbours microtubule- and ATP-binding activities. It comprises a catalytic core and an adjacent C-terminal neck region [2] . Kinesin undertakes one step per ATP hydrolysed [3] . The corresponding processive movement is driven by two alternate conformations of the two kinesin neck linkers (the ca . 15 amino acids C-terminal to the motor domain core), docked and undocked, in correlation with the nucleotide bound to each motor domain [4] , giving rise to a transport rate at the level of 100 steps per second [3] . To determine the mechanism for movement production, a detailed structural analysis of the kinesin in its different nucleotide states is required. Numerous X-ray structures of kinesins detached from their track protein are known; these kinesins are mostly bound to ADP (for example, see refs 5 , 6 , 7 ; for a review, see ref. 8 ) but in a few cases ATP-like structures have been determined [9] , [10] . There is also a recent structure of ATP-like kinesin bound to tubulin [11] (ATP-like complex). In addition, kinesin motor domains in all their nucleotide states, bound to microtubules, have been studied by cryo-electron microscopy (EM) at resolutions up to ca . 9 Å [12] , [13] , [14] , [15] . However, for a complete description of the kinesin nucleotide cycle, a high-resolution structure of the nucleotide-free kinesin bound to its track protein (nucleotide-free complex) is required. Because of this missing structure, open questions remain about critical features of the kinesin mechanism. One such feature is that neck linker docking, which initiates each step taken, only happens on ATP binding to the motor domain [4] . The related specific question concerns the structural changes caused in tubulin-bound kinesin on ATP binding that lead to neck linker docking and result in movement. So far, it has only been possible to define the mixed effects on the kinesin structure of tubulin and nucleotide binding [11] . The comparison of the atomic resolution structures of the nucleotide-free and ATP-like complexes would distinguish these effects and clarify how ATP binding initiates each step. A second critical feature is that in the absence of microtubules, motile kinesins are trapped in an ADP-bound state, thereby minimizing futile ATP hydrolysis. Trapping terminates on microtubule binding, which accelerates ADP release by several orders of magnitude [16] . The corresponding mechanism remains elusive [14] . The comparison of kinesin–ADP with a structure of nucleotide-free kinesin would define structural changes in the nucleotide site that lower the affinity for ADP. To address these issues, we have determined the structure of nucleotide-free kinesin bound to tubulin at 2.2 Å resolution and compared it with those of detached kinesin–ADP and of the complex of tubulin with kinesin–ADP-AlF 4 − (hereafter referred to as the ATP-like complex). These comparisons show that the kinesin structural changes along the nucleotide cycle are well described by rigid-body movements of three motor subdomains. As kinesin binds to tubulin, these movements distort the nucleotide-binding site and cause ADP release. The high-resolution structure we determined identifies the atomic interactions that are established in nucleotide-free kinesin by residues that interact with the nucleotide in kinesin–ADP. Our results also identify the interactions of ATP that cause subdomain movements resulting in the opening of a cavity in the motor core where the first residue of the neck linker gets buried, initiating neck-linker docking. In addition, our results suggest a connection between neck-linker docking and ATP hydrolysis. Therefore, the structure of the nucleotide-free complex has allowed us to establish the reciprocal relationship between neck-linker docking on the one hand and ATP binding and hydrolysis on the other hand. Taken together, our results clarify the link between the kinesin nucleotide cycle and movement. 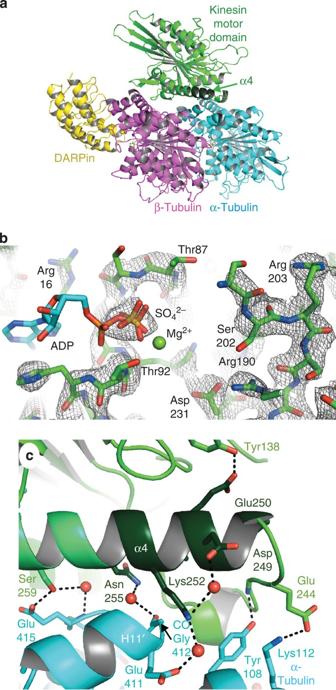Figure 1:The structure of nucleotide-free kinesin bound to tubulin. (a) Overview of the complex crystallized. (b) Two Fobs-Fcalc map (contoured at the 1σlevel) of the nucleotide-free complex centred at the nucleotide-binding site of (apo-) kinesin. ADP and Mg2+are from kinesin–ADP (1BG2) after superposition of the kinesin P-loop subdomains (seeFig. 2a) in these two structures. In the apo-kinesin nucleotide site, no water molecule has been identified but an SO42−ion that largely overlaps with the ADP β-phosphate and accounts for the observed electron density has been modelled. A stereo image of the electron density is presented inSupplementary Fig. 1. (c) The α4 N-terminal extension is stabilized both by direct and water (red spheres)-mediated interactions with α-tubulin and the motor domain core. The kinesin is in green with the extension of the α4 helix, which forms in all nucleotide states on binding to tubulin11,14, in darker green (as ina); α-tubulin is in cyan. All figures of structural models were generated with Pymol51. Structure of nucleotide-free kinesin in complex with tubulin We determined the structure of an apo-kinesin motor domain bound to tubulin ( Supplementary Table 1 ). For crystallization, the motor domain was truncated after the first amino acid of the neck linker, as this peptide has been shown to be disordered in nucleotide-free tubulin-bound kinesin [4] (this means that the construct crystallized comprises residues 1–325). Furthermore, tubulin was complexed to a designed ankyrin repeat protein (DARPin) [17] that prevents its assembly [18] ( Fig. 1a ). As expected, there is no nucleotide in the kinesin nucleotide-binding site ( Fig. 1b and Supplementary Fig. 1 ). Comparable to when ATP-like [11] , the kinesin in its nucleotide-free form is able to bind to curved tubulin, whereas it moves along microtubules in which tubulin is straight. Nevertheless, the structure of apo-kinesin in the nucleotide-free complex is very similar to that of apo-kinesin monomers that decorate microtubules [14] ( Supplementary Fig. 2 ). As in cryo-EM reconstructions of microtubule-bound kinesin motor domains [12] , [14] , the α4 helix at the interface with tubulin is longer at its amino-terminus than in detached kinesin–ADP; we find that similar to that in the ATP-like complex [11] , it is extended by 2.5 turns ( Fig. 1c ). Furthermore, we compared the overall conformations of curved and microtubular tubulin residues at the interface with the kinesin, as had been done in the case of the ATP-like complex. We found that they are highly similar, the root mean square deviation of the Cαs of tubulin residues at the interface with kinesin being 1.5 Å (34 Cαs compared). Local or overall variations in kinesin structure corresponding to these small differences at the surface of tubulin are not detected at the ca . 9 Å resolution of cryo-EM maps currently available [14] . Therefore, both the kinesin and its interface with tubulin are similar in the nucleotide-free complex and in a microtubule-decorating kinesin. Thus, the structure we determined, in comparison with those of the ATP-like complex [11] and of detached kinesin–ADP [5] , [6] , provides the basis for the identification of microtubule- and ATP-induced changes. Figure 1: The structure of nucleotide-free kinesin bound to tubulin . ( a ) Overview of the complex crystallized. ( b ) Two Fobs-Fcalc map (contoured at the 1 σ level) of the nucleotide-free complex centred at the nucleotide-binding site of (apo-) kinesin. ADP and Mg 2+ are from kinesin–ADP (1BG2) after superposition of the kinesin P-loop subdomains (see Fig. 2a ) in these two structures. In the apo-kinesin nucleotide site, no water molecule has been identified but an SO 4 2− ion that largely overlaps with the ADP β-phosphate and accounts for the observed electron density has been modelled. A stereo image of the electron density is presented in Supplementary Fig. 1 . ( c ) The α4 N-terminal extension is stabilized both by direct and water (red spheres)-mediated interactions with α-tubulin and the motor domain core. The kinesin is in green with the extension of the α4 helix, which forms in all nucleotide states on binding to tubulin [11] , [14] , in darker green (as in a ); α-tubulin is in cyan. All figures of structural models were generated with Pymol [51] . 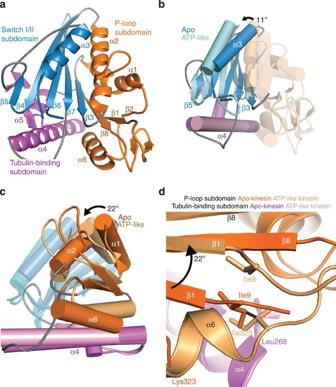Figure 2:Changes in tubulin-bound apo-kinesin on ATP binding. (a) The three subdomains whose movements account for structural changes during the nucleotide cycle. For clarity, the strands that are not part of the central β sheet are not labelled. The subdomains connecting loops are in grey. (b) The movement of the Switch I/II subdomain on ATP binding. In this and inc, the tubulin-binding blocks in ATP-like and in apo-kinesin have been superimposed and the subdomain that is not being compared is shown as a semi-transparent model. (c) The movement of the P-loop subdomain; for clarity, strands β1a–β1c, which are not part of the central β sheet, have been omitted. (d) The effect of the P-loop subdomain rotation on neck-linker docking. P-loop subdomains in ATP-like and apo-kinesin are presented following superposition of the tubulin-binding blocks. The location of the first neck-linker residue (Ile325) in ATP-like kinesin is occupied by Ile9 in nucleotide-free kinesin (the atoms linked by a black solid line are 1.2 Å away). As a consequence, in the nucleotide-free complex the kinesin polypeptide chain is disordered after Lys323. Full size image A remarkable property of the nucleotide-free complex is the plasticity of kinesin, which is notably more flexible than tubulin ( Supplementary Table 2 ). The kinesin atomic temperature factors increase gradually from its tubulin interface to its tubulin distal surface ( Supplementary Fig. 3 ). The kinesin temperature factors distribution in the nucleotide-free complex is unlikely to be due to the curvature of tubulin, as in the ATP-like complex [11] , in which tubulin is just as curved as in the nucleotide-free complex, temperature factors of the tubulin and kinesin partners are similar ( Supplementary Table 2 ). Instead, the flexibility seems specific to apo-kinesin, which is consistent with the notion that it is prone to denaturation [19] unless it is stabilized on strong binding to tubulin (or microtubules) in the rigor state. The mechanism by which ATP controls neck-linker docking The structure of the nucleotide-free complex was first compared with that of the ATP-like complex [11] . The comparison shows that the motor domain binds to tubulin through the same interface in both nucleotide states. However, because of the higher resolution of the nucleotide-free complex crystals diffraction and as the tubulin–kinesin interface is highly ordered, additional interactions mediated by trapped water molecules were identified in the structure determined in this work ( Fig. 1c ). The new structure differs from the structure of the ATP-like state by a considerable reorganization of the majority of the motor domain, as well as by local changes in the nucleotide-binding motifs (Switch1, Switch2 and the P-loop). The general reorganization of the motor is best described by relative rigid-body movements of three subdomains: a tubulin-binding subdomain that lies at the kinesin–tubulin interface (helices α4 and α5, the intervening L12 loop and strands β5a and β5b), a P-loop subdomain (constituted of both ends of the motor domain core—strands β1 and β2 of the core β sheet, helices α1 and α2 at the N-terminal end, and β8 and α6 at the C-terminal end) and a Switch I/II subdomain (β3–β7 and α3) ( Fig. 2a and Supplementary Fig. 4 ; for the nomenclature of secondary structure elements, see these figures and refs 5 , 20 ). When the kinesin tubulin-binding subdomains in the nucleotide-free and ATP-like complexes are superimposed, additional 11° and 22° rotations are required to superimpose the Switch I/II and P-loop blocks, respectively (root mean square deviation after superposition are 0.64 and 0.58 Å, over 84 and 111 Cαs, respectively) ( Fig. 2b,c and Supplementary Movie 1 ). Movements of these two subdomains also account for the other structural changes in the kinesin nucleotide/microtubule binding cycle ( Fig. 3 ) as well as for their functional consequences. In particular, when tubulin-binding subdomains in the nucleotide-free and detached ADP-bound kinesin are superimposed, the Switch I/II block is rotated 9° and the P-loop block is rotated 7° between the two structures. These rotations distort the nucleotide-binding site to cause ADP release (see ‘The acceleration of nucleotide release on tubulin binding’ in the Results section). Figure 2: Changes in tubulin-bound apo-kinesin on ATP binding . ( a ) The three subdomains whose movements account for structural changes during the nucleotide cycle. For clarity, the strands that are not part of the central β sheet are not labelled. The subdomains connecting loops are in grey. ( b ) The movement of the Switch I/II subdomain on ATP binding. In this and in c , the tubulin-binding blocks in ATP-like and in apo-kinesin have been superimposed and the subdomain that is not being compared is shown as a semi-transparent model. ( c ) The movement of the P-loop subdomain; for clarity, strands β1a–β1c, which are not part of the central β sheet, have been omitted. ( d ) The effect of the P-loop subdomain rotation on neck-linker docking. P-loop subdomains in ATP-like and apo-kinesin are presented following superposition of the tubulin-binding blocks. The location of the first neck-linker residue (Ile325) in ATP-like kinesin is occupied by Ile9 in nucleotide-free kinesin (the atoms linked by a black solid line are 1.2 Å away). As a consequence, in the nucleotide-free complex the kinesin polypeptide chain is disordered after Lys323. 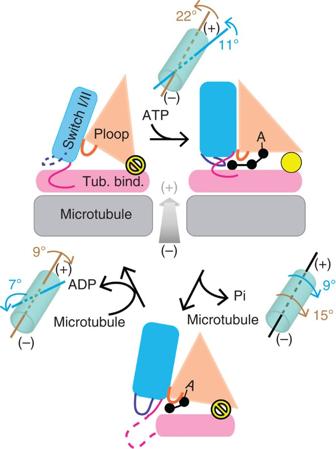Figure 3: Subdomains orientation changes along the kinesin mechanochemical cycle. The angles are those of the rotations needed to superimpose the P-loop (salmon, with the P-loop in orange) and Switch I/II (blue, Switch1/L9 in darker blue) subdomains, after the tubulin-binding blocks (pink) have been superimposed. The Switch2/L11 loop is in darker pink. The root mean square deviation of Cα positions after superposition are all smaller than 1 Å. The rotation axes are schematized taking the microtubule (depicted as a cylinder, with its polarity indicated) as a reference. Note that the rotations that relate subdomains in detached kinesin and in the ATP-like complex are around nearly parallel axes so that the three subdomains were not readily identified based on these two structures. The yellow disk indicates the status of the neck linker, which docks along with ATP binding but does not in the nucleotide-free state. After phosphate release and detachment from the microtubule, kinesin–ADP undergoes recovery to a state in which the neck linker undocks and becomes disordered, as schematized. Full size image Figure 3: Subdomains orientation changes along the kinesin mechanochemical cycle. The angles are those of the rotations needed to superimpose the P-loop (salmon, with the P-loop in orange) and Switch I/II (blue, Switch1/L9 in darker blue) subdomains, after the tubulin-binding blocks (pink) have been superimposed. The Switch2/L11 loop is in darker pink. The root mean square deviation of Cα positions after superposition are all smaller than 1 Å. The rotation axes are schematized taking the microtubule (depicted as a cylinder, with its polarity indicated) as a reference. Note that the rotations that relate subdomains in detached kinesin and in the ATP-like complex are around nearly parallel axes so that the three subdomains were not readily identified based on these two structures. The yellow disk indicates the status of the neck linker, which docks along with ATP binding but does not in the nucleotide-free state. After phosphate release and detachment from the microtubule, kinesin–ADP undergoes recovery to a state in which the neck linker undocks and becomes disordered, as schematized. Full size image The effect of ATP binding on the relative orientations of the Switch I/II and P-loop subdomains may be analysed as follows. In the ATP-like complex [11] , whereas the ADP moiety binds mostly to the P-loop subdomain, the γ-phosphate analogue and the nucleotide-bound Mg 2+ establish a network of interactions with the P-loop and with completely conserved residues in the Switch I/II subdomain (Ser201 and Ser202 in the Switch1 motif and Asp231 in the Switch2 motif) [9] , [10] , [11] . These interactions could not be made in the nucleotide-free complex ( Supplementary Fig. 5 ). Only following relative reorientation of the Switch I/II and P-loop subdomains can the interaction of Asp231 with two of the groups that coordinate Mg 2+ be established; this reorientation together with the new structure of the Switch1 loop allows Ser201 and Ser202 to interact with Mg 2+ as well as with the γ-phosphate analogue ( Supplementary Fig. 5 ). Therefore, ATP bridges the Switch I/II and P-loop blocks through the multiple simultaneous interactions it mediates, which favours the reorientation of the two subdomains. Another consequence of ATP binding to the tubulin-bound kinesin is the docking of the neck linker. For the neck linker to be docked, the side chain of its first residue (Ile325, highly conserved in kinesins) needs to be buried in a cavity in the kinesin motor domain core that is boxed in by Ile9 in the P-loop subdomain and three highly conserved residues (Ile265, Leu268 and Leu290) in the tubulin-binding subdomain ( Supplementary Fig. 6 ). In tubulin-bound kinesin this cavity is formed only in the ATP state, whereas it collapses in the apo state as the position of the first residue of the docked neck linker is largely occupied by the side chain of Ile9 ( Fig. 2d ). The residue at position 9 of the sequence is not as well conserved as the other residues that constitute the Ile325 cavity, but an isoleucine or a valine are most commonly found. Remarkably, in the recently determined rigor-like structure of the kinesin-3 KIF14 (ref. 21 ), the residue equivalent to Ile9 (a valine) is located as in the nucleotide-free complex and would interfere with neck-linker docking similarly to Ile9 in kinesin ( Fig. 2d ). Thus, taken together with structural evidence from the literature, our data lead us to propose that ATP binding triggers neck-linker docking by inducing the rotation of the P-loop subdomain. This will be further supported when additional structural data, for example, on apo-kinesin constructs with a longer neck linker, become available. Neck-linker docking gates the kinesin ATPase As mentioned above, when the neck linker is docked, its first residue (Ile325) would severely clash with Ile9 of the P-loop block in its nucleotide-free orientation ( Fig. 2d ), suggesting that neck-linker docking prevents the P-loop subdomain from rotating back from its ATP-like orientation towards the nucleotide-free one. As the structure of kinesin in the ATP-like complex is tuned for an efficient ATP hydrolysis chemical step [10] , [11] , this means that neck-linker docking locks the structure in an ATPase-competent state. Indeed, deleting the neck linker (yielding the 1–324 construct) decreased the microtubule-stimulated ATPase by 60-fold compared with the 1–349 monomeric construct, which comprises the full neck linker in addition to the motor domain core ( Table 1 ). Removal of the whole neck linker has been reported previously to have a substantial effect on microtubule-stimulated ATPase of another (+) end-directed kinesin, the kinesin-3 Kif1a [22] . We also found that incorporating the first residue of the neck linker (yielding the construct used for crystallization in this work) increased the ATPase rate by a factor of 20, the remaining difference from the 1–349 construct ( Table 1 ) being most likely due to the missing interactions mediated by the rest of the neck linker. These results strongly suggest that Ile325 contributes significantly to positioning the P-loop subdomain for efficient ATP hydrolysis when the neck linker is docked. Table 1 Microtubule-stimulated ATPase kinetic parameters of truncation and substitution mutants of the kinesin motor domain. Full size table Our model leads to another prediction concerning the shortened constructs (1–324 and 1–325). As the neck linker is disordered [4] and does not interfere with the P-loop subdomain in the nucleotide-free complex, the model predicts that ADP release should be much less affected than the ATPase chemical step in these constructs and become non-rate limiting. Indeed, we found that the maximum rates of microtubule-stimulated Mant-ADP release from both constructs (52.9±7.4 and 43.0±3.3 s −1 , respectively; see Supplementary Fig. 7 ) are much higher than their respective k cat kinetic constants and similar to the k cat kinetic constant of the 1–349 construct ( Table 1 ). Interestingly, the ATPase of a triple mutant comprising residue changes I325A/K326A/N327A is unaffected [23] . This result is well accounted for by the structures, as the Cβ of residue 325 in a docked neck linker clashes with Ile9 in apo-kinesin ( Fig. 2d ), so that the ATPase-efficient positioning of the P-loop subdomain is still maintained in this triple mutant. To attenuate the clash between Ile9 and Ile325, we mutated the latter residue to a glycine in the 1–349 construct. This should lessen the interference of residue 325 with the nucleotide-free orientation of the P-loop subdomain and lead to a much decreased ATPase activity. This is what we observed: the ATPase activity of the I325G mutant was decreased by 27-fold ( Table 1 ). This decrease of the ATPase activity could also be due to a general destabilization of the kinesin structure. If this was the case, one would expect ADP to be less tightly bound in the mutated protein. However, such is not the case: the rate of spontaneous ADP release from the I325G mutant is very similar to that from the parent construct (0.015 s −1 versus 0.025 s −1 ), implying that the effect of the I325G mutation on the ATPase rate is not due to an overall destabilization of the kinesin. Taken together, our results therefore suggest that when the neck linker is docked, the interference of Ile residues at positions 9 and 325 of the sequence locks the P-loop subdomain in its ATPase-competent orientation. Our results are also consistent with a kinetic model of kinesin motility, which concluded that the rear head of a kinesin dimer, to which the neck linker is docked, has a much higher ATPase activity than the front head, in which the neck linker is undocked [24] . They strongly support the proposal that neck-linker docking gates the ATPase activity of the kinesin motor domain. The acceleration of nucleotide release on tubulin binding Next, we compared the structures of kinesin in the tubulin:apo-kinesin complex and of detached kinesin–ADP [5] . As mentioned above, when kinesin binds to tubulin, the α4 helix extends by 2.5 turns ( Fig. 1 ) at its N-terminal end, the corresponding residues being prone to disorder in detached kinesin (for example, see refs 5 , 6 ). When kinesin–ADP binds to tubulin and if the α4 helix lengthened without additional changes, severe clashes would arise between the extension and the rest of the motor domain. In particular, Glu250, Asn253 and Ile254 in the extension would strongly clash with Tyr138 and Leu139 in the turn connecting strands β4 and β5 of the kinesin central sheet ( Fig. 4a ) and with Arg203 in the Switch1 motif ( Supplementary Fig. 8 ). In apo-kinesin, these clashes are avoided through two main changes. Most of the Switch1-containing L9 loop is disordered, instead of forming a short helical segment as in kinesin–ADP [5] ( Supplementary Fig. 8 ). In addition, the Switch I/II subdomain rotates by 7° with respect to the tubulin-binding block ( Fig. 3 ) so that Tyr138 makes a hydrogen bond with Glu250 and Leu139 does not interfere with the α4 extension ( Fig. 4a ). This rotation is accompanied by a P-loop subdomain movement that allows the extensive interactions of the Switch I/II and P-loop blocks to be maintained (the buried surface area at their interface is larger than 2,000 Å 2 in all nucleotide states). These conformational changes of the kinesin on tubulin binding reorganize the nucleotide-binding site, as detailed below. 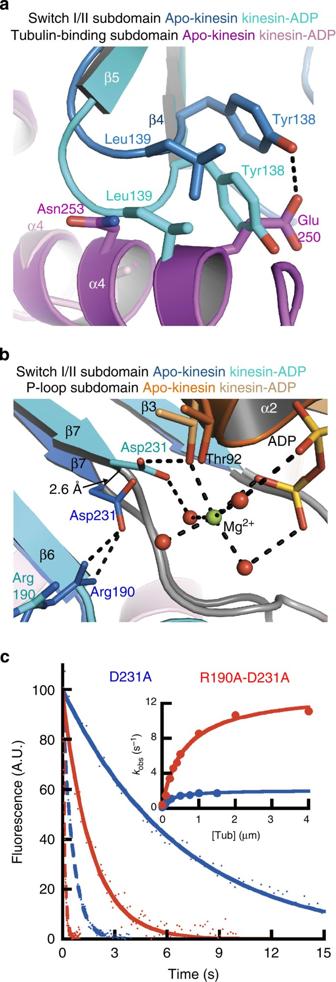Figure 4:Changes between detached kinesin–ADP and tubulin-bound apo-kinesin. (a) The α4 extension is not compatible with the structure of the β4–β5 turn in kinesin–ADP. Kinesin–ADP5has been superimposed on nucleotide-free kinesin in the tubulin complex by overlapping common α4 residues (residues 255 to 270). Residues of the β4-β5 turn that clash with residues in the α4 extension are presented. (b) Changes in the nucleotide-binding site caused, on tubulin binding, by the rotations of the Switch I/II and P-loop subdomains. The P-loop subdomains have been superimposed to show the changes in the interactions of Asp231 with the Mg2+-coordinating ligands. For clarity, the Mg2+coordinating water molecules are the only ones presented. (c) Kinetics of mant-ADP release from the D231A and R190A-D231A kinesin mutants. Fluorescence variations on release from the D231A (blue) and R190A-D231A (red) kinesins in the absence of microtubules (solid lines) or stimulated by 1 μM microtubular tubulin (dashed lines) are shown (10% of the experimental points are displayed) after normalization following subtraction of a linear component due to photobleaching. The line is the fit by an exponential decay function. The inset tocgives the variation ofkobsas a function of microtubular tubulin concentration for both mutants. Figure 4: Changes between detached kinesin–ADP and tubulin-bound apo-kinesin . ( a ) The α4 extension is not compatible with the structure of the β4–β5 turn in kinesin–ADP. Kinesin–ADP [5] has been superimposed on nucleotide-free kinesin in the tubulin complex by overlapping common α4 residues (residues 255 to 270). Residues of the β4-β5 turn that clash with residues in the α4 extension are presented. ( b ) Changes in the nucleotide-binding site caused, on tubulin binding, by the rotations of the Switch I/II and P-loop subdomains. The P-loop subdomains have been superimposed to show the changes in the interactions of Asp231 with the Mg 2+ -coordinating ligands. For clarity, the Mg 2+ coordinating water molecules are the only ones presented. ( c ) Kinetics of mant-ADP release from the D231A and R190A-D231A kinesin mutants. Fluorescence variations on release from the D231A (blue) and R190A-D231A (red) kinesins in the absence of microtubules (solid lines) or stimulated by 1 μM microtubular tubulin (dashed lines) are shown (10% of the experimental points are displayed) after normalization following subtraction of a linear component due to photobleaching. The line is the fit by an exponential decay function. The inset to c gives the variation of k obs as a function of microtubular tubulin concentration for both mutants. Full size image In kinesin–ADP [5] , similar to tubulin:kinesin–ATP [11] , the nucleotide is bound by interactions with P-loop subdomain residues and by the completely conserved Switch2 N-terminal residue, Asp231. This residue makes hydrogen bonds with two of the groups that coordinate the ADP-bound Mg 2+ ion [22] , [25] , the Thr92 (in the P-loop) hydroxyl and a water molecule oxygen atom. As Asp231 belongs to the Switch I/II subdomain ( Supplementary Fig. 4 ), the movements of the Switch I/II and P-loop blocks during the transition to the nucleotide-free state displace Asp231 by 2.6 Å with respect to the P-loop subdomain ( Fig. 4b ). As a consequence, the simultaneous interactions of ADP-Mg 2+ with the P-loop subdomain and Asp231 witnessed in detached kinesin cannot be maintained in tubulin-bound kinesin, where ADP release is substantially accelerated. These observations suggest that the tight binding of ADP in detached kinesin is, at least partially, due to the interactions made by Asp231. To quantify the contribution of Asp231 to ADP trapping, we mutated it to alanine in the 1–349 construct and recorded the spontaneous ADP release from this mutant. We found that the release rate (0.15±0.01 s −1 , see Fig. 4c ) is substantially faster than that of the parent construct (0.025±0.01 s −1 ), confirming a role for the Asp231 interactions with Mg 2+ in ADP binding in tubulin-unbound kinesin. To evaluate the effect of the overall structural changes that accompany tubulin binding, we also measured microtubule-stimulated nucleotide release from the D231A mutant. The rate increases as a function of the tubulin concentration, its maximum value (1.9±0.1 s −1 , see Fig. 4c ) being similar to the ATPase rate ( Table 1 ), meaning that nucleotide release limits the ATP hydrolysis rate in this mutant. The rate for microtubule-stimulated ADP release from D231A is much slower than that from the parent monomeric construct, which is at least as fast as the ATPase rate (~50 s −1 , similar to previously measured values [3] ). A molecular explanation for this difference is provided below. Asp231 makes a salt bridge with Arg190 in the nucleotide-free complex ( Fig. 4b ). Therefore, mutating it to an alanine leaves the positive charge of the arginine unbalanced. To eliminate a possible effect of this altered charge distribution, we produced the R190A-D231A double mutant of the 1–349 construct and measured the rate at which it releases ADP. The basal rate is accelerated compared with the D231A mutant (to 0.6±0.1 s −1 ) as is the microtubule-stimulated rate (13±0.5 s −1 , Fig. 4c ), which still limits the ATPase rate ( Table 1 ). Not unexpectedly, as kinesin is tuned for efficient microtubule-stimulated ADP release, the rate displayed by the double mutant is still slower than that by the 1–349 construct. The most probable explanation is that the interactions made by Asp231 and Arg190 in the nucleotide-free microtubule-bound kinesin also contribute to accelerating ADP release. To sum up, the overall structural changes caused by the re-orientations of the motor subdomains and, in particular, the change of Asp231 location lead to microtubule-stimulated ADP release from kinesin. In this study, we have determined the structure of nucleotide-free kinesin bound to tubulin. Comparison of this structure to that of ATP-like kinesin bound to tubulin [11] has led to the identification of three kinesin motor subdomains whose movements account for kinesin structural changes along the nucleotide cycle ( Fig. 3 ). Of these, only the tubulin-binding subdomain had been identified for its most part, using two approaches: by alanine-scanning mutagenesis of the kinesin [26] and by structural studies using X-rays and cryo-EM, in particular of a fast kinesin-1 from Neurospora crassa [7] . The three subdomains scheme differs from that deduced from cryo-EM studies, which depicted changes as rotations of the entire catalytic core of the motor domain, relative to the fixed α4 helix [14] . The identification of the subdomains was made possible because of the resolution of the structures we have determined and because of the large differences between tubulin-bound ATP-like [11] and apo-kinesin ( Fig. 3 ). The distinction of three motor subdomains is also of interest in the context of the comparison of the kinesin and myosin families of motor proteins. The structural similarity of the kinesin motor domain core to the myosin catalytic domain surrounding the nucleotide was noticed when the first kinesin structure was determined [5] and suggested a common evolutionary ancestor [27] . However, whereas a substantial rearrangement of the core β sheet has been seen in nucleotide-free myosins [28] , [29] , [30] , such a change has long been looked for unsuccessfully in kinesins [31] and the resulting distortion was observed only recently in the KIF14–ADP structure [21] . Our data demonstrate that the core β sheets in nucleotide-free and kinesin–ATP are distorted in respect to each other ( Supplementary Fig. 9a and Supplementary Movie 2 ). Remarkably, in both myosins and kinesin, the central β sheet is similarly partitioned into two subdomains (the Switch I/II and P-loop blocks in kinesin, which correspond to the upper 50 kDa and to the N-terminal myosin domains, respectively Supplementary Fig. 9b ), and distorts when the subdomains change their relative orientation. This further strengthens the parallel between the two families of proteins, highlighting that they interact with the nucleotide through a common mechanism. The distinct insertions between the structural elements of the myosin and kinesin catalytic cores allow them to adapt to their different cycles of interaction with their tracks and to the different relations between their nucleotide and mechanical cycles [31] . Our results clarify the mechanism for nucleotide release on tubulin binding, a mechanism that had remained elusive so far [32] . They suggest an important role of the Mg 2+ ion in the binding of ADP to detached kinesin. Interestingly, Mg 2+ is an inhibitor of ADP release from detached Kif1a [22] . The change of Asp231 location in microtubule-bound kinesin is expected to disrupt Mg 2+ binding and to suppress its inhibitory effect. Indeed, Mg 2+ has no inhibitory effect on ADP release from microtubule-bound Kif1a [22] . A mechanism similarly involving the disruption of the Mg 2+ coordination has been demonstrated for the exchange-factor-mediated dissociation of GDP from the P21 ras GTPase [33] , [34] . The high-resolution structure we determined also identifies a salt bridge established in nucleotide-free kinesin between Asp231 and Arg190, two residues that are, respectively, fully and highly conserved in kinesins. This salt bridge stabilizes the nucleotide-free structure, compensating at least in part for the interactions made between Asp231 and the nucleotide in kinesin–ADP. As we propose that nucleotide release results from relative movements of the Switch I/II and P-loop motor subdomains, interactions that hinder or alter these movements are predicted to influence ADP release. Such interactions were identified between the motor and the inhibitory tail domains in a kinesin [35] , [36] . Taken together with the structure of tubulin-bound apo-kinesin, mutants analysis and inhibition data strongly argue that microtubule-stimulated ADP release is due to a distortion of the nucleotide binding site that, in particular, disrupts the Mg 2+ coordination. This distortion is caused by microtubule-induced relative movements of the Switch I/II and P-loop subdomains. The structural changes of tubulin-bound kinesin on ATP binding are also accounted for by our scheme. The direct effect of ATP binding is to bridge the P-loop and the Switch I/II subdomains ( Supplementary Fig. 5 ), following which the orientations of these two blocks change. Therefore, neck-linker docking is an indirect consequence of ATP binding, as the former only becomes possible following rotation of the P-loop subdomain ( Fig. 2d ). Indeed, kinetic studies have shown that neck-linker docking follows ATP binding [37] . We also found that neck-linker docking gates the ATPase activity, because its first residue (Ile325) latches the motor domain in a hydrolysis-efficient conformation. This is also consistent with previous studies, suggesting a direct feedback of neck-linker docking to the catalytic site [38] . Importantly, the connection between neck-linker docking and ATPase efficiency reduces the probability that in a dimer the microtubule-bound motor hydrolyses ATP before its companion head has been propelled in the direction of the movement. This contributes to the large processivity and thermodynamic efficiency of kinesin. In summary, our work has enlightened three important aspects of motile kinesins mechanism that concern the three main reactions of their nucleotide cycle: the acceleration of nucleotide release on microtubule binding, the connection between ATP binding and neck-linker docking, and that between neck-linker docking and ATP hydrolysis. Taken together, these results set up a general framework for understanding the mechanism of kinesin-1. Because of the conservation of the sequences as well as of the regions involved in movement generation, the structural scheme, which we described for kinesin-1 mechanism, is likely to apply to other (+) end-directed kinesins. Proteins The monomeric kinesins used in this study (constructs 1–349, 1–325 or 1–324, and the D231A, R190A-D231A and I325G mutants based on the 1–349 construct) were obtained by standard molecular biology techniques from a cys -light version of human kinesin, which has been shown to have kinetic properties that are identical to those of kinesin [4] . They were produced in BL21 cells grown in 2YT medium. When A600 reached 0.7–0.8, protein expression was induced with 0.3 mM isopropyl β- D -1-thiogalactopyranoside at 18 °C overnight. Cells were suspended in 10 ml g −1 of wet cells of 50 mM Mes-Na pH 6.0, 1 mM MgCl 2 , 0.5 mM EGTA, 10 μM ATP, 1 mM dithiothreitol (DTT) (Buffer A) to which 1 mM phenylmethylsulfonyl fluoride and protease inhibitors mix (complete EDTA free, Roche Applied Science) were added. Cells were lysed using a French press and cells debris were removed by centrifugation at 20,000 g for 20 min at 4 °C. DNAse (1 μg ml −1 ) was added for 15 min at room temperature, the kinesin-containing solution was centrifuged at 30,000 g for 45 min at 4 °C and the supernatant was collected. Purification was performed on a Äkta Purifier system using two ion-exchange chromatography steps. First a Hitrap SP FF column (GE Healthcare) in Buffer A, eluting with a 0–30% Buffer B (Buffer A+1 M NaCl) gradient. Second a Mono Q (GE Healthcare) column in a buffer containing 50 mM Tris-HCl pH 7.0, 1 mM MgCl 2 , 0.5 mM EGTA, 10 μM ATP, 1 mM DTT and 10% sucrose. The column was eluted with a 10–40% gradient of the Tris buffer to which 1 M NaCl had been added. The protein was then concentrated, quantified according to its optical density at 280 nm and stored in liquid N 2 until use. Tubulin was purified by two polymerization/depolymerization cycles in a high-molarity buffer [39] and stored in liquid N 2 in 50 mM Mes-K pH 6.8, 33% glycerol, 0.25 mM MgCl 2 , 0.5 mM EGTA, 0.1 mM GTP until use. Before use, an additional microtubule assembly/disassembly cycle was performed to remove any non-functional protein. The disassembly step was carried out in 15 mM Mes-K pH 6.8, 0.5 mM MgCl 2 , 0.5 mM EGTA. Tubulin concentration was determined spectrophotometrically using an extinction coefficient at 278 nm of 1.2 mg −1 ml −1 cm −1 assuming the molecular mass of the heterodimer is 100 kDa [40] . The DARPin was expressed in XL1-Blue cells grown in 2YT medium. When A600 reached 0.7–0.8, protein expression was induced with 0.5 mM isopropyl β- D -1-thiogalactopyranoside for 4 h at 37 °C. Cells were suspended in 10 ml g −1 of wet cells of 50 mM Tris, pH 8 (4 °C), 1 mM MgCl 2 , 10 mM imidazole, 0.3 mg ml −1 lysozyme and protease inhibitor mix (complete EDTA free, Roche Applied Science). Cells were lysed by sonication and cells debris were removed by centrifugation at 20,000 g for 20 min at 4 °C. Purification was performed on a Äkta Purifier system using a Histrap column (GE Healthcare). Eluted protein was subjected to size-exclusion chromatography on a Superdex 75 column equilibrated with 20 mM potassium phosphate pH 7.2, 1 mM MgCl 2 , 0.5 mM EGTA, 100 mM KCl. D1 concentration was estimated by ultraviolet absorption using an extinction coefficient of 6,990 M −1 cm −1 derived from the peptide sequence using the ProtParam webserver ( http://web.expasy.org/protparam ). To prepare the complex with apo-kinesin, kinesin was incubated with tubulin–DARPin in a 1:1 ratio, then desalted through a PD10 column (GE healthcare) to remove unbound nucleotide. We checked that this procedure yields nucleotide-free kinesin by separating any remaining ADP from the tubulin nucleotides on a Mono Q column (GE Healthcare) after trifluoroacetic acid denaturation of the proteins. ADP was then quantified based on comparison of the peak areas with those of an equimolar ADP:GDP:GTP sample of known concentration. ATPase The ATPase activities of kinesin were measured at 25 °C by using an enzyme-coupled assay [41] in a buffer consisting of 20 mM Pipes pH 6.8, 1 mM MgCl 2 , 0.5 mM EGTA, 1 mM DTT and 1 mM ATP. The enzymes and reagents for the assay (phosphoenolpyruvate, NADH, pyruvate kinase and lactate dehydrogenase) were from Sigma-Aldrich. Varying amounts of docetaxel-stabilized microtubules were added before addition of the kinesin (0.5 μM) and 20 μM docetaxel was supplemented in the buffer to stabilize microtubules. The variations of the stimulated ATPase rate as a function of microtubule concentrations were analysed according to the Michaelis–Menten equation to yield k cat and K M . ADP release As a means to evaluate the ADP release rate, kinesin constructs were loaded with Mant-ADP and the fluorescence decrease associated with dissociation from kinesin was monitored using a SX20 Stopped-Flow Spectrometer at 25 °C. Specifically, kinesin was incubated for 30 min on ice with a threefold excess of Mant-ADP in a buffer consisting of 25 mM Pipes-Na pH 6.8, 2 mM MgCl 2 , 1 mM EGTA, 1 mM DTT, following which the kinesin was desalted using a Micro Bio-spin 6 column (BioRad) to remove unbound nucleotide. Next, 0.5 μM kinesin was mixed with an equal volume of buffer supplemented with 1 mM ADP, with or without microtubules, and the fluorescence intensity (excitation at 355 nm) was recorded using a 400 nm long-pass filter. We verified that superimposable time courses were obtained with 2 mM ADP or with 1 mM ATP (as used by others [42] , [43] , [44] ), confirming that the recorded process truly represents the dissociation of Mant-ADP, which kinetically limits the binding of ADP (and of ATP) in all the conditions tested. Data were fitted to determine an observed rate constant of the fluorescence decay, k obs . For microtubule-stimulated Mant-ADP release, the variation of k obs as a function of the tubulin concentration was fitted with a hyperbolic curve to determine the stimulated release kinetic constant k off . Crystallization and structure determination The apo-kinesin–tubulin–DARPin complex was crystallized at 293 K by vapour diffusion with a crystallization buffer consisting of 30% (W/V) polyethylene glycol 5000 monomethyl ether, 0.1 M Mes-K pH 6.5 and 0.2 M ammonium sulphate. The crystal was harvested in the same solution supplemented with 20% glycerol, then flash-frozen in liquid nitrogen. A 2.2 Å data set was collected at 100 K at the Proxima1 beam line (Soleil Synchrotron, Saint Aubin, France). It was processed with XDS [45] and SCALA [46] . The structure was solved by molecular replacement with PHASER [46] using tubulin-DARPin (pdb id 4DRX) and kinesin–ADP (1BG2) as starting models. The structure was refined with Buster [47] with iterative model building in Coot [48] . The final model includes 1,331 residues, 99.2% of which are in favoured and allowed regions of the Ramachandran plots, while 0.8% are outliers, as evaluated with MolProbity [49] . Data processing and refinement statistics are summarized in Supplementary Table 1 . Identification of the kinesin subdomains Kinesin subdomains that are invariant in the nucleotide-free and the ATP-like complexes were identified with the programme RAPIDO [50] using a ‘low limit’ value of 1. How to cite this article: Cao, L. et al . The structure of apo-kinesin bound to tubulin links the nucleotide cycle to movement. Nat. Commun. 5:5364 doi: 10.1038/ncomms6364 (2014). Accession codes: Coordinates and structure factors have been deposited with the Protein Data Bank (accession code: 4LNU ).